A DNA tweezer-actuated enzyme nanoreactor The functions of regulatory enzymes are essential to modulating cellular pathways. Here we report a tweezer-like DNA nanodevice to actuate the activity of an enzyme/cofactor pair. A dehydrogenase and NAD + cofactor are attached to different arms of the DNA tweezer structure and actuation of enzymatic function is achieved by switching the tweezers between open and closed states. The enzyme/cofactor pair is spatially separated in the open state with inhibited enzyme function, whereas in the closed state, enzyme is activated by the close proximity of the two molecules. The conformational state of the DNA tweezer is controlled by the addition of specific oligonucleotides that serve as the thermodynamic driver (fuel) to trigger the change. Using this approach, several cycles of externally controlled enzyme inhibition and activation are successfully demonstrated. This principle of responsive enzyme nanodevices may be used to regulate other types of enzymes and to introduce feedback or feed-forward control loops. Nature has evolved a myriad of enzymes to catalyze chemical reactions that are vital to the metabolism and reproduction of living systems [1] . The ability to regulate those enzyme's activities in response to cellular environmental conditions (for example, substrate levels, stimulants, etc.) is critical to many metabolic functions [2] , [3] . Scientists are currently interested in finding ways to mimic enzyme regulatory circuitry outside of the cell [4] , [5] , not only to increase our knowledge of cellular metabolism but also so that we may create man-made nanoreactors that have potential utility in applications ranging from diagnostics to the production of high-value chemicals [6] , [7] , [8] and smart materials [9] . DNA nanostructures are promising scaffolds for use in the organization of molecules on the nanoscale because they can be engineered to site-specifically incorporate functional elements in precise geometries [10] , [11] , [12] and to enable nanomechanical control capabilities [13] , [14] . Examples of such structures include autonomous walkers [15] , [16] , nanotweezers [17] , [18] , [19] , [20] and nanocages for controlled encapsulation and payload release [21] , [22] . New protein–DNA conjugation chemistries make it possible to precisely position proteins and other biomolecules on DNA scaffolds [23] , generating multi-enzyme pathways with the ability to modulate intermolecular interactions and the local environment [24] , [25] , [26] , [27] , [28] , [29] , [30] . Taking advantage of these features, we exploit a DNA tweezer nanostructure to actuate the activity of a glucose-6-phosphate dehydrogenase (G6pDH)/NAD + enzyme/cofactor pair. Here, the enzyme and cofactor are displayed from different arms and actuation of enzyme function is achieved by switching between open and closed states to spatially separate the enzyme/cofactor pair for inhibition, or bring the pair together for activation, respectively. Design of DNA tweezers The mechanics of the DNA tweezer-regulated enzyme nanoreactor are shown in Fig. 1a . The design and construction of the nanotweezers, with ~14-nm long arms, are based on a previous report [17] . A 25-nucleotide (nt) single-stranded DNA (ssDNA) oligomer (5′-TTTGCGTAAGACCCACAATCGCTTT-3′) connects the ends of the tweezer arms and serves as a structural regulatory element to control the state of the tweezers (please see Supplementary Fig. S1 for detailed sequences). In the initial closed state the regulatory oligomer is designed to adopt a ‘GCG’ stem-loop hairpin structure that holds the two arms of the tweezers close together. The average distance between the arms in the closed state is ~6.9 nm, according to fluorescence energy transfer measurements (FRET) [31] , [32] ( Supplementary Fig. S2 ). The open state is achieved by disrupting the hairpin via hybridization of a complementary set strand to it, thereby generating a rigid ~16-nm long double-helical domain between the ends of the tweezer arms. To switch back to the closed state a fuel strand that is fully complementary to the set strand is introduced to the system, releasing the regulatory oligomer to a hairpin by a strand-displacement mechanism [33] . The open and closed tweezers were also characterized with AFM as shown in Supplementary Fig. S3 . 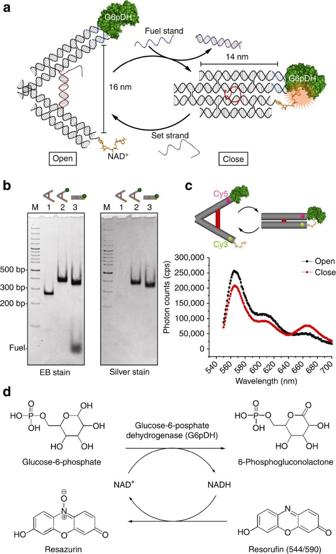Figure 1: Design and characterization of G6pDH/NAD+-assembled DNA tweezers. (a) Schematic illustration of the mechanics of the DNA tweezer-regulated enzyme nanoreactor: a regulatory oligomer (shown in red) is designed to adopt a ‘GCG’ stem-loop hairpin structure that holds the two arms of the tweezers close together. The addition of a set strand (complementary to the regulatory loop shown in red) to the tweezer structure results in the formation of a DNA double helix between the tweezer arms that separates the G6pDH and NAD+enzyme/cofactor pair (open state). Displacement of the set strands from the regulatory loop by fuel strands leads to the active state (closed) in which G6pDH and the cofactor NAD+are in close proximity. (b) Characterization of the fully assembled tweezers structures: left—ethidium bromide-stained PAGE gel for detecting DNA; right—the same gel visualized by silver stain for detecting proteins. Lane 1: open tweezers with NAD+attached by a poly(T)20linker; lane 2: open tweezers assembled with G6pDH; lane 3: closed tweezers assembled with G6pDH. All structures were purified using biotin–avidin affinity resins. (c) FRET measurement experiment (Cy3/Cy5 dyes) to characterize the open and closed states of the tweezers. (d) Detection of enzymatic activity in the G6pDH/NAD+-assembled tweezers using a phenazine methosulfate (PMS)/resazurin-coupled assay: NAD+is first reduced to NADH by G6pDH. Next, PMS catalyzes electron transfer from NADH to resazurin producing a strongly fluorescent resorufin with an emission of maximum ~590 nm. Figure 1: Design and characterization of G6pDH/NAD + -assembled DNA tweezers. ( a ) Schematic illustration of the mechanics of the DNA tweezer-regulated enzyme nanoreactor: a regulatory oligomer (shown in red) is designed to adopt a ‘GCG’ stem-loop hairpin structure that holds the two arms of the tweezers close together. The addition of a set strand (complementary to the regulatory loop shown in red) to the tweezer structure results in the formation of a DNA double helix between the tweezer arms that separates the G6pDH and NAD + enzyme/cofactor pair (open state). Displacement of the set strands from the regulatory loop by fuel strands leads to the active state (closed) in which G6pDH and the cofactor NAD + are in close proximity. ( b ) Characterization of the fully assembled tweezers structures: left—ethidium bromide-stained PAGE gel for detecting DNA; right—the same gel visualized by silver stain for detecting proteins. Lane 1: open tweezers with NAD + attached by a poly(T) 20 linker; lane 2: open tweezers assembled with G6pDH; lane 3: closed tweezers assembled with G6pDH. All structures were purified using biotin–avidin affinity resins. ( c ) FRET measurement experiment (Cy3/Cy5 dyes) to characterize the open and closed states of the tweezers. ( d ) Detection of enzymatic activity in the G6pDH/NAD + -assembled tweezers using a phenazine methosulfate (PMS)/resazurin-coupled assay: NAD + is first reduced to NADH by G6pDH. Next, PMS catalyzes electron transfer from NADH to resazurin producing a strongly fluorescent resorufin with an emission of maximum ~590 nm. Full size image DNA-conjugated protein and NAD + Next, G6pDH was conjugated to a ssDNA (5′-TTTTTCCCTCCCTCC-3′) using well-developed chemical methods [24] . The complementary anchor strand was displayed from one of the tweezer arms to capture the DNA-modified G6pDH via sequence-specific hybridization. The other arm of the DNA tweezers was functionalized with an amino-modified NAD + molecule [34] . The detailed conjugation chemistry and characterization are described in Supplementary Figs S4–S8 . Characterization of enzyme-tweezer assembly The G6pDH/NAD + -assembled tweezer complex was characterized by native polyacrylamide electrophoresis (PAGE) as shown in Fig. 1b . The protein-bound (~100 kD for G6pDH) [35] DNA tweezers exhibited reduced mobility in the PAGE gel due to the relatively higher molecular weight. In addition, the closed-state tweezers migrated slightly faster than the open-state tweezers due to their more compact conformation. The identity of each band in the gel was verified by ethidium bromide [36] and silver staining [37] , where ethidium bromide preferentially bound to the DNA and the metallic silver solution of the protein. The expected band shifts were confirmed by both staining methods. A high yield of enzyme-bound tweezers is visible in the gel images, with evidence of successful switching between open and closed states. As shown in Fig. 1c , we also characterized the conformational state of the fully assembled tweezers using FRET between Cy3/Cy5 dye pairs. Here, the end of one of the tweezer arms was labeled with Cy3 and the other with Cy5. The closed tweezers exhibited a lower Cy3 signal and a higher Cy5 signal due to relatively efficient energy transfer between the fluorophores. As shown in Fig. 1d , a resazurin-coupled assay was used to evaluate the activity of the tweezer-bound G6pDH/NAD + pair. The assay involves the phenazine methosulfate-catalyzed reduction of resazurin to resorufin by NADH, as evidenced by the production of a strong fluorescence signal (excitation ~544 nm, emission ~590 nm) [38] . To remove any unassembled enzymes and minimize the background signal all tweezer constructs were purified by biotin-affinity resin treatment ( Supplementary Fig. S9 ). Optimization of the activity of enzyme-assembled tweezers In an effort to optimize the activity of the G6pDH/NAD + -assembled tweezers, the NAD + cofactor was attached to the tweezers by a single-stranded poly thymidine (T) linker. As shown in Fig. 2a , we investigated the dependence of the length of the poly (T) linker on the activity of the G6pDH/NAD + -assembled tweezers (raw activity traces shown in supplementary Fig. 10 ). Most tweezers were correctly assembled and able to open and close as characterized by native PAGE in Fig. 2c . A small amount of aggregation (<10%) of the tweezer constructs was observed due to DNA–DNA stacking. The activities of both the open and closed tweezers improved as the length of the linker was increased from 0 to 20 nts (~30 nm in linear length), presumably due to the enhanced flexibility of the longer linkers. Further increasing the linker length from 20 nts to 40 nts (~60 nm in linear length) did not improve the enzyme activity, but rather resulted in a slight decrease. We also evaluated the ability of the tweezers to modulate enzymatic activity by determining the relative level of enhancement of the closed state compared to the open state. As shown in Fig. 2b , >5.5-fold activity enhancement was observed for closed tweezers with no linker, or with a short poly (T) 3 linker. As the length of the linker increased, the enhancement in the activity of the closed tweezers compared to the open tweezers gradually decreased. Tweezers with a relatively long poly (T) 40 linker exhibited less than four-fold activity enhancement. This is likely because longer linkers increase the accessibility of NAD + to G6pDH even in the open state, thereby reducing the ability of the tweezers structure to modulate enzyme activity. We selected a poly (T) 20 linker for attachment of the NAD + cofactor to the tweezers, which yielded more than three-fold higher enzymatic activity than tweezers with no linker, and maintained greater than five-fold activity enhancement of closed tweezers compared to open ones. In this way, we were able to sustain adequate enzyme activity while also preserving the regulatory capacity of the tweezers. 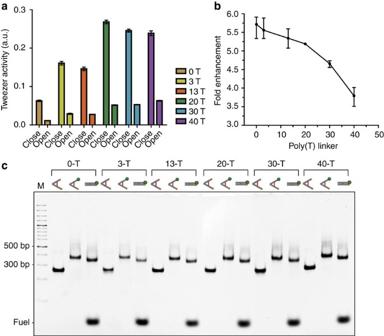Figure 2: Optimization of the NAD+linker length for tweezer activity and actuation. (a) The activities of open and closed tweezers as a function of poly(T) linker length. (b) Enhancement of closed tweezers compared to opened tweezers as a function of poly(T) linker length. (c) Native PAGE characterization of all DNA tweezers with different poly(T) linker length. Slight aggregations of tweezers were observed due to DNA–DNA stacking. Figure 2: Optimization of the NAD + linker length for tweezer activity and actuation. ( a ) The activities of open and closed tweezers as a function of poly(T) linker length. ( b ) Enhancement of closed tweezers compared to opened tweezers as a function of poly(T) linker length. ( c ) Native PAGE characterization of all DNA tweezers with different poly(T) linker length. Slight aggregations of tweezers were observed due to DNA–DNA stacking. Full size image Regulatory cycling of the enzyme-assembled tweezers We further examined the ability of the G6pDH/NAD + tweezers to withstand several cycles of on/off enzyme activity. In Fig. 3a , we present a native PAGE gel that demonstrates the ability of the assembled tweezers to switch between open and closed states nine times while maintaining their structural integrity. Additional cycles are limited by the accumulation of large amounts of set and fuel strands. We also monitored the real-time opening and closing of the tweezers by labeling the tweezer arms with Cy3 and Cy5 FRET dyes, respectively. As shown in Fig. 3b , Cy3 emitted less fluorescence in the closed state due to energy transfer to Cy5, whereas Cy5 exhibited higher emission under the same conditions. The gradual decrease in the intensity of Cy3 fluorescence observed over time can be attributed to photo bleaching. Real-time kinetic analysis revealed that the tweezers switch from open to closed states very quickly, with all tweezers transformed within a few seconds (too fast to measure the kinetic constant accurately). However, the kinetics of switching from the closed to open state is much slower, with a first-order kinetic constant of ~0.0025±0.0003, s −1 . The rate constants corresponding to switching from the closed to open state gradually increased as the cycle number increased: ~0.0051, s −1 for the second cycle, ~0.0054, s −1 for the third cycle, and 0.0071, s −1 for the fourth cycle ( Supplementary Figs S11 and S12 ). It is likely that the relatively sluggish process of tweezer opening is due to the slow hybridization of the set strand to the self-folded hairpin structure connecting the tweezer arms and the subsequent disruption of the rather stable hairpin structure. The results in Fig. 3c demonstrate the ability of the DNA tweezer structure to regulate G6pDH activity by switching between open and closed states (raw activity traces shown in Supplementary Fig. S13 ). The tweezers were able to actuate the on/off enzyme activity eight times in 200 min, with the closed state producing five-fold higher enzymatic activity on average than the open state. 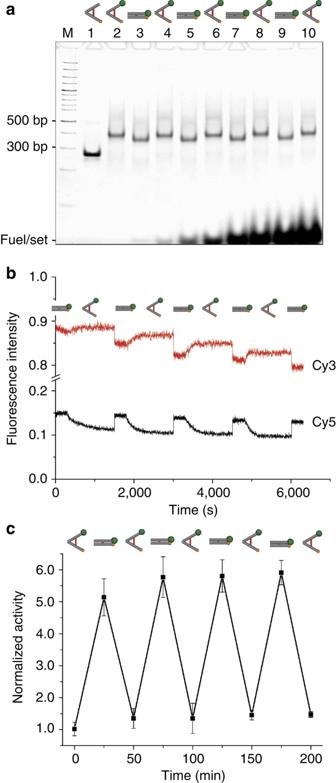Figure 3: Regulatory cycling of the G6pDH/NAD+-assembled tweezers. Four cycles of conformational and functional transition were measured and analyzed using (a) native PAGE, (b) real-time FRET and (c) enzymatic assay. Cycles were initiated in the open state, and for each conformational change 50% excess fuel or set strands were added. All the enzyme activities were normalized to the activity of initial open tweezers. Figure 3: Regulatory cycling of the G6pDH/NAD + -assembled tweezers. Four cycles of conformational and functional transition were measured and analyzed using ( a ) native PAGE, ( b ) real-time FRET and ( c ) enzymatic assay. Cycles were initiated in the open state, and for each conformational change 50% excess fuel or set strands were added. All the enzyme activities were normalized to the activity of initial open tweezers. Full size image In conclusion, we have designed and constructed a DNA tweezer-like nanostructured enzyme system with the ability to turn on and off the activity of a G6pDH/NAD + enzyme/cofactor pair by means of nanomechanical control. In the open state the tweezer conformation inhibits the activity of the G6pDH/NAD + enzyme/cofactor pair by holding the molecules apart, while in the closed state the close proximity of the pair results in greatly enhanced activity. We successfully demonstrated several cycles of enzyme inhibition and activation in response to external stimuli (regulatory DNA strands). With additional developments in DNA–protein/cofactor attachment chemistry it should be possible to regulate other types of enzymes and to introduce feedback or feed-forward control loops. In the future it may be feasible to develop responsive enzyme nanodevices as highly specific chemical amplifiers in diagnostic applications or as biocatalysts in the production of high-value chemicals and smart materials. Preparation of enzyme-assembled DNA tweezers N -Succinimidyl 3-(2-pyridyldithio)-propionate was used to crosslink G6pDH with a 5′ thiol-modified oligonucleotide [24] . Detailed protein–oligo conjugation protocol is shown in Supplementary Methods . An amino-modified NAD + analog was conjugated to a 5′ amine-modified oligonucleotide using a disuccinimidyl suberate linker on an anion-exchange DEAE–Sepharose resin. Detailed conjugation protocol and NAD activity characterization are shown in Supplementary Fig. S14 and Supplementary Methods . DNA tweezers were prepared in 1 × TAE/Mg 2+ buffer (40 mM Tris, 20 mM acetic acid, 2 mM EDTA and 12.5 mM magnesium acetate, pH 8.0) at a final concentration of 0.5 μM, except for the set strand and the strand conjugated to NAD + , both of which had final concentrations of 0.75 μM. All samples were annealed in an Eppendorf Mastercycler. The temperature steps in the annealing protocol were as follows: first the temperature was decreased from 90 °C to 72 °C over 10 min (2 °C min −1 ), then decreased from 68 °C to 24 °C over 60 min (1.25 °C min −1 ), then held constant at 4 °C ( Supplementary Table S1 ). Tweezers concentration was determined by the estimated extinction coefficient at 260 nm ( Supplementary Table S2 ). A three-fold molar excess of oligonucleotide-conjugated G6pDH was added to the pre-annealed tweezer structures and mixed completely. Protein assembly was performed using an annealing protocol in which the temperature was gradually decreased from 37 °C to 10 °C over a period of 1 h and then held constant at 4 °C using an established procedure [24] . Excess G6pDH-WN1 was removed by affinity of the biotin-labeled tweezers using monomeric avidin resin (Pierce). Enzymatic assay of G6pDH/NAD + tweezers In all, 100 nM G6pDH/NAD + -assembled DNA tweezers were assayed with 100 μl of 1 mM glucose-6-phosphate, 1 mM phenazine methosulfate and 500 μM resazurin. Magnesium ion was removed from the sample solution by biotin purification to avoid the formation of double-stranded DNA/Mg 2+ complexes that quench resorufin fluorescence ( Supplementary Figs S15,S16 ). The activity of the enzyme-bound DNA tweezers was measured by monitoring the fluorescence increase at 590 nm that results from the reduction of reasazurin to fluorescent resorufin by NADH. For more detailed information, please see Supplementary Methods . How to cite this article: Liu, M. et al. A DNA tweezer-actuated enzyme nanoreactor. Nat. Commun. 4:2127 doi: 10.1038/ncomms3127 (2013).